Dynamic reassortments and genetic heterogeneity of the human-infecting influenza A (H7N9) virus Influenza A (H7N9) virus has been causing human infections in China since February 2013, raising serious concerns of potential pandemics. Previous studies demonstrate that human infection is directly linked to live animal markets, and that the internal genes of the virus are derived from H9N2 viruses circulating in the Yangtze River Delta area in Eastern China. Here following analysis of 109 viruses, we show a much higher genetic heterogeneity of the H7N9 viruses than previously reported, with a total of 27 newly designated genotypes. Phylogenetic and genealogical inferences reveal that genotypes G0 and G2.6 dominantly co-circulate within poultry, with most human isolates belonging to the genotype G0. G0 viruses are also responsible for the inter- and intra-province transmissions, leading to the genesis of novel genotypes. These observations suggest the province-specific H9N2 virus gene pools increase the genetic diversity of H7N9 via dynamic reassortments and also imply that G0 has not gained overwhelming fitness and the virus continues to undergo reassortment. Since 30 March 2013, when the first laboratory-confirmed case of the novel avian influenza A (H7N9) virus infection of humans was formally reported [1] , there have been a total of 139 confirmed human infections in 11 provinces of China, with 45 deaths (as of 6 November 2013) ( http://www.moh.gov.cn ; http://www.who.int/csr/don/2013_11_06/en/index.html ). The outbreak has been controlled by integrative measures including the closedown of the wet markets in the affected areas. A single reoccurring case was just reported on 15 October, in Zhejiang Province, China. Until now, there have been no confirmed cases of human-to-human transmission, and most infected humans had a history of contact with poultry or of having visited a wet market [2] , [3] , [4] , [5] , [6] , although suspected human-to-human transmission has been described [7] . Our previous analyses on the first released virus genomes proposed that this virus might have emerged from at least four origins by means of genetic reassortment [3] . Aside from the haemagglutinin (HA) and neuraminidase (NA) genes that might have originated from wild birds along the East Asian flyway, the six internal genes may have been derived from at least two separate H9N2 lineages, which have been circulating within Chinese poultry populations for several years. Interestingly, the virus of this outbreak exhibits relatively diversified features according to previous studies [3] . In particular, the virus strain, A/Shanghai/1/2013, showed some differences to the other viruses in both the phylogenies and specific amino-acid substitutions in the HA and NA proteins [1] , [3] , [4] , [6] , [8] , [9] . In addition, the NP gene presented a certain divergence, and the strain A/Shanghai/1/2013 is clustered together with A/chicken/Shanghai/C1/2012(H9N2), rather than the other two H7N9 isolates [3] . Recently, the PB2 , PB1 , PA and M genes have also been found to form at least two clusters in the phylogenetic trees [10] , [11] . All these suggest that the H7N9 viruses of this outbreak might be diversified far beyond what we observed from preliminary studies, and consequently a more comprehensive study was called for to uncover the veil of the H7N9 virus. To further shed light on the genetic features of this novel virus, we performed extensive surveillance in six cities of Jiangsu and Zhejiang provinces, including Nanjing, Suzhou, Wuxi, Zhenjiang, Xuzhou and Hangzhou, which were the majorly affected areas in this outbreak. Twenty H7N9 virus strains from patients, poultry and wet markets were isolated and sequenced. 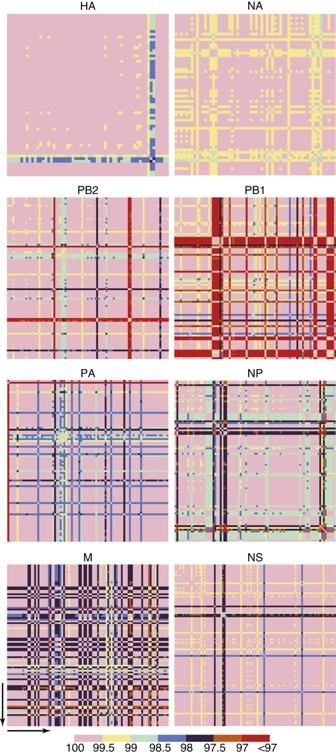Figure 1: Matrices showing gene identities of H7N9 virus genes. The identity ranges are indicated by different colours. The arrows represent the isolation date, from the earliest to the latest. Together with the H7N9 virus genomes available in the GISAID and GenBank databases, we collected sequences from a total of 109 H7N9 isolates, of which 89 had their full-length genome sequenced ( Supplementary Table 1 ). These viruses were isolated from 10 provinces, with 38 from human and 51 from poultry or the environment. Strikingly, the sequence analysis and phylogenies illustrate a high degree of diversity in the internal genes of the H7N9 viruses, represented by 27 genotypes. Furthermore, the genealogical inferences reveal that genotype G0 accounts for the spread of this virus, and that both inter-province and intra-province transmissions have contributed to the genesis of novel virus genotypes. Moreover, the two major genotypes, G0 (A/Anhui/1/2013-like viruses) and G2.6 (A/chicken/Shanghai/S1078/2013-like viruses), are found to have co-circulated among poultry. These findings imply that the H7N9 virus continues to evolve, and that the dynamic reassortments with H9N2 viruses play an essential role in the genesis of novel reassortants. The internal genes of H7N9 exhibit a great diversity We first performed sequence alignment and pairwise comparison of all high-quality H7N9 virus genes. Surprisingly, pairwise alignments showed that the internal genes of H7N9 were much more divergent than the HA and NA genes ( Table 1 ), which encode the surface proteins and could be more divergent [12] , [13] , [14] . HA and NA genes of the H7N9 viruses showed ~2% mismatches for the most divergent sequence pair, while >3% mismatches were observed for the internal genes. The mean values of the sequence identity also showed that the HA and NA genes of the H7N9 viruses were more conserved than internal genes. When we transformed the identity matrix of each viral gene into a heat map, it was obvious that the internal genes showed more heterogeneous patterns, in which there were more genes possessing greater diversity ( Fig. 1 ). Moreover, the divergent patterns showed by the internal genes existed throughout the outbreak, seemingly having little correlations with the isolation date. Table 1 Sequence identity of human influenza virus isolates of different outbreaks. Full size table Figure 1: Matrices showing gene identities of H7N9 virus genes. The identity ranges are indicated by different colours. The arrows represent the isolation date, from the earliest to the latest. Full size image We further compared the H7N9 viruses with the highly pathogenic H5N1 influenza viruses and the pandemic H1N1 (pH1N1). In particular, we chose the H5N1 viruses causing the outbreak in Vietnam and Thailand in 2004 (Clade 1), those in Egypt in 2006 (Clade 2.2), and the pH1N1 viruses in North America and in China ( Table 1 ). These outbreaks, like the H7N9 outbreak, were the first introduction to each region and had not experienced antigenic shift in the first season [15] , [16] , [17] . For the 2004 Vietnam–Thailand H5N1 outbreak, HA was the most diversified gene. Moreover, the mean identity of each internal gene was also greater than those of HA and NA. In the H5N1 outbreak in Egypt in 2006, both the HA and NA were distinctly more divergent than internal genes. Similar results of more conserved internal genes were also observed in the pH1N1 outbreaks, although only ~1% differences over the whole genome were found in both of the North American and Chinese data sets ( Table 1 ). All these observations were different from that we found in the H7N9 outbreak. However, when we examined the sequences of the H5N1 outbreak in Vietnam and Thailand in 2005, we obtained similar results to those observed in H7N9, in that internal genes presented more diversified features than surface genes ( Table 1 ). These viruses were the descendants of the 2004 Vietnam–Thailand outbreak and also evolved within local poultry. The sequence differences, especially the internal genes, were much greater than those of the 2004 Vietnam–Thailand outbreak, suggesting that these viruses might have undergone rapid genetic reassortments. It was generally believed that the surface proteins encountered greater positive selection pressures and thus changed faster than the internal genes [12] , [13] , [14] , especially when an influenza virus outbreak occurred in a naive population, such as the H5N1 and pH1N1 ( Table 1 ), and when generally few genotypes co-circulated [15] , [16] , [17] . It was thought that only when an influenza virus has evolved within a local region over a few seasons would internal gene reassortments become more frequent for better adaptation, resulting in the heterogeneity of the internal genes ( Table 1 ) and the prosperity of genotypes [15] , [18] , [19] . Specific to this H7N9 outbreak, the combination of the surface proteins is new to both human and poultry in China. However, the feature of the gene diversity resembled influenza virus having evolved longer periods within one region. Phylogenetics classifies internal genes into varied clades We then reconstructed phylogenetic trees for all eight viral genes using the maximum likelihood method. From the phylogenetic trees, the HA and NA genes were clustered together, implying that they might be derived from a single origin, respectively ( Supplementary Fig. 1 ). However, in the phylogenetic trees constructed using the six internal genes, the H7N9 strains could be grouped into more than one cluster, with one major cluster and at least one minor cluster ( Fig. 2 and Supplementary Fig. 2 ). In particular, the NS gene, which has been reported to form a single cluster in previous analyses, was found to form at least two clusters for the first time. Generally, the major clades included the majority of the H7N9 sequences, and sequences from the majority of the human isolates fell within each major clade. In the minor clades, the majority of isolates were from poultry/environment with only a few human isolates. Furthermore, closely related poultry H9N2 strains fell within most minor clades ( Supplementary Fig. 2 ). These H9N2 virus strains were isolated from chickens from the same province or adjacent provinces, such as Shanghai, Jiangsu, Shandong, and so on. Interestingly, none of the closely related H9N2 strains were found within each major clade, although a few H9N2 strains were found at the root of some of the major clades, such as the PA and NP genes. 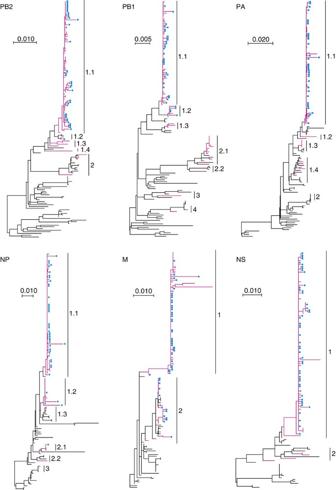Figure 2: Phylogenetic trees of the internal genes estimated using RAxML under the GTRGAMMA model. The branches in magenta represent the H7N9 viruses and those in black represent the H9N2 viruses. The human isolates were labeled by cyan dots. The clades and the assigned numbers were labeled aside. Figure 2: Phylogenetic trees of the internal genes estimated using RAxML under the GTRGAMMA model. The branches in magenta represent the H7N9 viruses and those in black represent the H9N2 viruses. The human isolates were labeled by cyan dots. The clades and the assigned numbers were labeled aside. Full size image Varied genotypes coexisted during the H7N9 outbreak To better display the diversity of the H7N9 viruses, we assigned genotypes for each H7N9 virus based on the clades from the phylogenetic analysis ( Fig. 3a , Supplementary Table 2 ). In general, viruses with all internal genes belonging to the major clade (Clade 1.1 or Clade 1) were assigned as genotype G0. The viruses within the G1 genotypes possess one internal gene distinct from G0 by the phylogenetic classification; the G2 series genotypes possess two distinct internal genes; and so on, with the viruses of the G6 series of genotypes having all six internal genes different from those of G0. Within each series, distinct genotypes were assigned if the internal genes of these viruses were different. Based on this rule, a total of 7 series and 27 distinct genotypes were designated ( Fig. 3a , Supplementary Table 2 ). Among them, G0 consisting of 40 isolates (22 human and 18 poultry/environmental) was the most dominant genotype, with one of the first isolates, A/Anhui/1/2013 (AH/1), as the representative strain. The second most dominant genotype series was G2, with a total of 23 isolates (5 human and 18 poultry/environment). 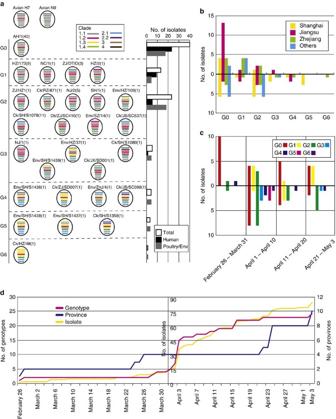Figure 3: Genotypic analysis of H7N9 viruses. (a) Proposed genotypes for the novel H7N9 viruses based on the phylogenies estimated using the internal genes. Genes in different clades were labeled with different colours. The representative strain is on the top of each cartoon and is followed by the total number of isolates in parenthesis. The abbreviations of the strains can be found inSupplementary Table 2. The chart on the right side represents the numbers of each genotype series. (b) Genotype distribution by region. Theyaxis denotes the number of isolates. The upper part illustrates human isolates and the lower part illustrates poultry/environmental isolates. (c) Genotype distribution by period. The upper part illustrates human isolates and the lower part illustrates poultry/environmental isolates. (d) Cumulative curves of the H7N9 isolates, genotypes and provinces. AH: Anhui; Ck: chicken; Env: environment; HZ: Hangzhou; JS: Jiangsu; JX: Jiangxi; NC: Nanchang; NJ: Nanjing; RZ: Rizhao; SH: Shanghai; SZ: Suzhou; ZJ: Zhejiang; ZnJ: Zhenjiang. Figure 3: Genotypic analysis of H7N9 viruses. ( a ) Proposed genotypes for the novel H7N9 viruses based on the phylogenies estimated using the internal genes. Genes in different clades were labeled with different colours. The representative strain is on the top of each cartoon and is followed by the total number of isolates in parenthesis. The abbreviations of the strains can be found in Supplementary Table 2 . The chart on the right side represents the numbers of each genotype series. ( b ) Genotype distribution by region. The y axis denotes the number of isolates. The upper part illustrates human isolates and the lower part illustrates poultry/environmental isolates. ( c ) Genotype distribution by period. The upper part illustrates human isolates and the lower part illustrates poultry/environmental isolates. ( d ) Cumulative curves of the H7N9 isolates, genotypes and provinces. AH: Anhui; Ck: chicken; Env: environment; HZ: Hangzhou; JS: Jiangsu; JX: Jiangxi; NC: Nanchang; NJ: Nanjing; RZ: Rizhao; SH: Shanghai; SZ: Suzhou; ZJ: Zhejiang; ZnJ: Zhenjiang. Full size image In humans, G0 acts as the dominant genotype, with G1, G2 and G3 existing at lower frequency. None of the G4, G5 and G6 isolates were observed in humans based on current surveillance data ( Fig. 3a ). However, in poultry and environment, G0 and G2 account for the majority of isolates, and all seven genotype series were observed. We then investigated the genotype distribution across province ( Fig. 3b ). For human isolates, G0 was dominant in Shanghai and Jiangsu, whereas G0 and G1 were equal in Zhejiang. However, for the poultry/environmental isolates, G2 was the most prevalent genotype series in Jiangsu, while G0 and G2 were equally dominant in Shanghai and Zhejiang. When the genotype distribution by isolation date was examined, we found that G0 was dominant in every period in human isolates, although G1, likely to be the reassortant derived from G0, was comparable during the days with the highest isolates (1 April to 10 April), and the period from 21 April to 3 May ( Fig. 3c ). Nevertheless, in poultry/environment, both G0 and G2 were the dominant genotypes. It should be noted that genotype G2.6, represented by A/Chicken/Shanghai/S1078/2013 (Ck/SH/S1078), accounted for nearly half (11/23) of the G2 series viruses. Additionally, we drew the accumulative curves to show the increase in the isolates and genotypes during the virus spreading ( Fig. 3d ). Only viruses with detailed isolation date were used. By 26 March, H7N9 viruses have been spread into four provinces, and 1 week after, the genotypes began to increase dramatically. The number of genotypes tended to reach a plateau on 16 April in these four provinces (Shanghai, Anhui, Jiangsu and Zhejiang). After 20 April, the viruses had spread into more provinces, and the number of genotypes also increased. The accumulation curves implicated that the increase in genotypes was relative to inter-province and intra-province transmissions. H7N9 diversity increases through virus transmissions In order to discern the relationship between the genetic diversity and virus transmission, we further performed the genealogical analysis to characterize the migration dynamics of the H7N9 viruses, applying a similar strategy as used in the study of the global migration of human influenza A/H3N2 (ref. 20 ). We classified the NA gene sequences into four groups according to the isolation provinces: Shanghai, Jiangsu, Zhejiang and the surrounding provinces (including Anhui, Shandong, Henan, Jiangxi, Taiwan, Fujian and Guangdong provinces) ( Fig. 4a ). We first tested the population differentiation of each region by using the fixation index ( F ST ) [21] , which is commonly used to quantify the genetic isolation among regions. On average, genetic diversity among contemporaneous sequences is greater between provinces, π b =2.90 (2.88, 2.99), than within provinces, π w =2.48 (2.46, 2.49). Therefore, F ST , quantified as ( π b − π w )/ π b , equals to 0.145 (0.142, 0.148) indicating genetic isolation among the provinces in this analysis. (Detailed information is given in Supplementary Table 3 .) Then we estimated the migration rates among these regions by using the Migrate [22] . The results revealed that the emigration rates from Shanghai, Jiangsu and Zhejiang to the other provinces were much higher ( Fig. 4b , Supplementary Tables 4 and 5 ), suggesting that the H7N9 viruses were transmitted to these provinces from Shanghai, Jiangsu and Zhejiang. This is in accordance with the epidemiological findings. In addition, only migrations from Shanghai to Jiangsu and Zhejiang were observed, but not the reverse directions. Migration of the viruses among Jiangsu, Zhejiang and the other provinces was also observed ( Fig. 4b ). This indicates that Shanghai is likely to have been the source of the virus, which then spreads to the surrounding provinces, and Jiangsu, Zhejiang and the other provinces where frequent virus transmissions, most likely through poultry transportations, also occurred. 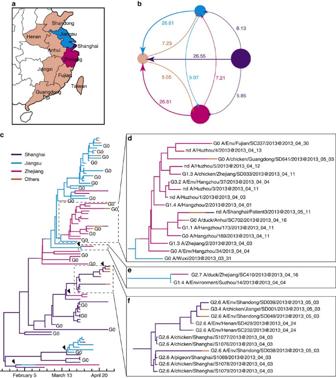Figure 4: Genealogical analysis of H7N9 viruses. (a) Map to show the geographical distribution of the provinces. (b) Migration rates between Shanghai, Jiangsu, Zhejiang and the remaining provinces. The colours were the same as ina. The area of each circle represents the centrality of each region in the migration network. The values represent the migration events per lineage per year. (c) Genealogy of the H7N9 viruses estimated using the NA gene sequences. Viruses of G0 were labeled. Arrowheads indicated the potential events of genotype change by inter-province transmission. (d,e) Representative clades to show genotype expansion through intra-province (d) and inter-province transmission (e). (f) Representative clade to show the spread of Ck/SH/S1078-like viruses (G2.6). The virus name, isolation date and genotype were labeled. nd: genotype not determined due to incomplete viral genome. Figure 4: Genealogical analysis of H7N9 viruses. ( a ) Map to show the geographical distribution of the provinces. ( b ) Migration rates between Shanghai, Jiangsu, Zhejiang and the remaining provinces. The colours were the same as in a . The area of each circle represents the centrality of each region in the migration network. The values represent the migration events per lineage per year. ( c ) Genealogy of the H7N9 viruses estimated using the NA gene sequences. Viruses of G0 were labeled. Arrowheads indicated the potential events of genotype change by inter-province transmission. ( d , e ) Representative clades to show genotype expansion through intra-province ( d ) and inter-province transmission ( e ). ( f ) Representative clade to show the spread of Ck/SH/S1078-like viruses (G2.6). The virus name, isolation date and genotype were labeled. nd: genotype not determined due to incomplete viral genome. Full size image To investigate the relationship between the migration dynamics of the viruses and genetic diversity of the internal genes, a detailed genealogical history of the human-infecting H7N9 virus population was reconstructed ( Fig. 4c ). In the virus genealogy, contacts between regions would produce migration events, indicated as shifts in colour. Then we mapped the genotype information of the H7N9 viruses on the virus genealogy ( Fig. 4c ). From the genealogical tree, we observed first that most viruses located at the trunk of the genealogy belonged to G0, implying that G0 might be responsible for the wide spread of the viruses and secondly that inter-province migration of the viruses led to not only the spread of G0 but also the genesis of novel genotypes ( Fig. 4c–f , Supplementary Fig. 3 ). The novel genotypes generated by inter-province transmission included G2.7, G3.1, G3.4, G4.2 and G6, although these observations may be due to the lack of surveillance. All viruses of these minor genotypes were terminal nodes in the genealogy and were not found to spread to other regions. We also observed that the continued circulation of the viruses within a local region (intra-province transmission) also increased the genetic diversity of the viruses. For example, genotypes G1.3, G1.4 and G3.2 in Zhejiang Province were most likely to be the result of the reassortment of G0 after introduction from Jiangsu Province (Wuxi City) ( Fig. 4d ). Moreover, we noticed that genotype G2.6 (the Ck/SH/S1078-like virus) circulating within poultry/environment formed a separated lineage in the genealogical tree ( Fig. 4f ). Originating from Shanghai, it appears that this genotype of viruses has spread to poultry in both Shandong and Henan. The fact that the internal genes of the H7N9 viruses possess higher diversity than the surface protein-encoding genes has raised the curiosity of the evolutionary traits of this pathogen. This strange phenomenon is most likely due to the use of the H9N2 internal gene cassette, which might have given the H7N9 viruses the ability to easily survive in poultry. The diversity of the internal genes is also well displayed in the phylogenetic trees, as the H7N9 internal genes clustered distinctly within the H9N2 lineages. Within most minor H7N9 clades, closely related H9N2 virus strains could be observed. Nevertheless, for the major clade of each phylogenetic tree, no H9N2 sequence was found to have fallen within the clade. One interpretation is the insufficient surveillance. However, another interpretation could be that the H7N9 virus had adopted the less prevalent H9N2 internal genes, and that the combination of these less prevalent genes might endow the H7N9 virus better fitness to poultry. However, it is still unknown whether there exists an H9N2 virus using this set of internal genes, as it is unlikely to exhibit fitness in poultry. The estimation of the most recent common ancestor for each virus gene suggested that the H7N9 viruses reassort sequentially [3] , [11] . Therefore, the recruitment of the internal genes of the H7N9 viruses from H9N2 seems far more complicated than expected. From the genotypic view, H7N9 has achieved a remarkable diversity in ~3 months. Since several genotypes have been shown to differ widely —for example, G6 has all internal genes different from G0—the H7N9 viruses might not have originated from a single genotype. In human isolates, G0 acted as the major genotype, while the G1 series (close relatives to G0) was less dominant, and no G4–G6 series genotypes were found in human isolates. This distribution of genotypes implies that the human isolates may have originated from a single genotype (most possibly G0), and that G0 possesses certain fitness in humans. The tuning of G0 has also created several reassortants capable of infecting humans, although these reassortants have as yet not showed better fitness for humans than G0. Meanwhile, among the poultry/environmental isolates, all series of genotypes were observed, and G0, together with G2.6, acted as the dominant genotypes co-circulating within poultry. So far, the G2.6 virus has not been identified as being able to infect humans, although it possesses the same receptor-binding pocket as G0 that had the potential to bind to human receptors. Surveillance has showed that the G2 series became more prevalent in poultry after 20 April, and the spread of G2 viruses deserves more attention. The migration dynamics and genealogy inferred by NA gene analysis have defined a map of virus transmission and proposed Shanghai as the epicentre of this H7N9 outbreak. Viruses in the other provinces were most probably transferred through poultry transportations, in accordance with surveillance data. The reason for using the NA gene sequences, instead of HA , to infer the migration dynamics and virus genealogy lies in that the majority of the antigenic sites located in HA and HA is responsible for the recognition and attachment to host receptors. Therefore, a number of factors drive the evolution of HA, including but not limited to migration. Analysis of H7N9 transmission by genotypes reveals the G0 viruses to be located along the trunk of the genealogy. This suggests that G0, the dominant genotype, was responsible for the spread of this virus, which is consistent with the surveillance evidence that found G0 in most provinces. Meanwhile, the G2.6 viruses may act as another important transmission pathway, which has spread out to a few provinces in poultry ( Fig. 4e ). In addition, as it seems that poultry are not infected as virus carriers, the G2.6 transmission pathway might have escaped surveillance. By now, no other genotype has spread to other provinces, and the according viruses only appeared at terminal nodes of the genealogic tree ( Supplementary Fig. 3 ). In addition, both the accumulative curves ( Fig. 3d ) and the genealogy revealed that both inter-province and intra-province transmissions of the H7N9 virus would contribute to the increase in genotypic diversity. These imply that control of virus transmission would dramatically reduce its genetic diversity. Based on the observations mentioned above, we proposed a dynamic reassortment model for the H7N9 virus evolution ( Fig. 5 ). Following the H7 and N9 viruses entering into the H9N2 virus hosts, the viruses began to recruit internal genes to adapt to the new hosts. Here the less prevalent H9N2 internal genes provided better fitness to the H7N9 viruses and finally formed the ancestor of the H7N9 viruses. It is likely that due to the complication of the reassortments, more than one genotype of H7N9 viruses would have originated. Thus, G0 along with several other genotypes were generated with G0 exhibiting the greatest fitness. In addition to reassortment within local H9N2 gene pool, the H7N9 virus, facilitated by poultry transportations, was transmitted to varied poultry populations and fell into different H9N2 gene pools. Within these gene pools, the virus experienced further genetic reassortments and dynamically generated more diversified genotypes of which some occasionally infected humans. It should be noted that the vast diversity of genotypes implicates that the virus is still undergoing genetic tuning. 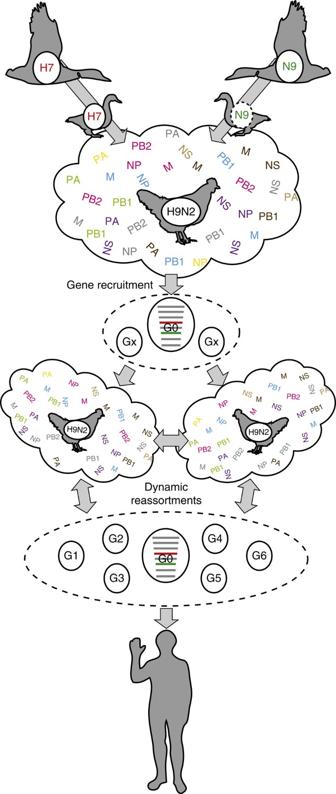Figure 5: Schematics illustrating the formation and dynamic reassortments of the H7N9 influenza viruses. Migratory bird, duck, chicken and human involved in the H7N9 emergence were shown in cartoons. Dashed circle of N9 represents the uncertainty of N9 in ducks due to the lack of surveillance data. Coloured internal gene names in clouds represent diversified H9N2 gene pools. Figure 5: Schematics illustrating the formation and dynamic reassortments of the H7N9 influenza viruses. Migratory bird, duck, chicken and human involved in the H7N9 emergence were shown in cartoons. Dashed circle of N9 represents the uncertainty of N9 in ducks due to the lack of surveillance data. Coloured internal gene names in clouds represent diversified H9N2 gene pools. Full size image The H7N9 virus has been demonstrated to possess the potential for human-to-human transmission [7] , [23] , and structural resolution of the HA protein showed the binding affinity to mammalian receptors [8] . However, the rare human-to-human transmission might be limited by the combination of internal genes, which may affect the fitness to mammalian hosts. As H7N9 was of low pathogenicity in poultry and as these dynamic reassortments were unnoticed until human infections occurred, it is unpredictable whether a ‘super’ reassortant with greater fitness to mammalian hosts could appear in the future. Hence, extensive surveillance of poultry production and transportation is urgently called for, especially for those H9N2 viruses that harboured genetic signatures for mammalian adaptation. Virus isolation and genome sequencing Specimens were maintained in a viral-transport medium. The specimens were inoculated and grown in 9- to 11-day-specific pathogen-free embryonated chicken eggs for 48–72 h at 35 °C. Viral RNA was extracted from sample using the RNeasy Mini Kit (QIAGEN, Germany). Standard reverse transcription–PCR was performed with the primers specific for influenza A virus using PrimeScript II 1st Strand cDNA Synthesis Kit (TaKaRa, Japan) and Ex-taq HS (TaKaRa). Double-strand cDNA was synthesized with Sequenase 2.0 (USB). Sequencing libraries were prepared using the Nextera XT DNA Sample Preparation Kit (Illumina). Samples were pooled together and then run on Illumina MiSeq platform to generate150-bp paired-end reads. The amplified PCR products were also sequenced on ABI 3730 automatic DNA analyzer (Life Technologies) with ABI BigDye Terminator V3.1 cycle sequencing kit (Life Technologies) at Sangon (Shanghai, China). Calculation of the percent identity of influenza viruses The percent identity of each virus genes was calculated by using the needle program in the EMBOSS package [24] . Data sets were obtained from the Influenza Virus Resource [25] and GISAID databases. For H5N1 data sets, we applied the database search with region/country and year as criteria. For 2009 North American pH1N1 viruses, we first searched H1N1 viruses with the following criteria: ‘host=human, year=2009, month=4–6, country=USA, Canada or Mexico’ then reconstructed the HA and NA phylogenetic trees with neighbour-joining methods, and excluded the seasonal flu viruses. Strain A/California/4/2009 was used as reference strain of pH1N1. For China pH1N1 viruses, we searched database with ‘host=human, year=2009, month=9–11, country=China’, and used neighbour-joining tree to exclude seasonal influenza viruses as well. Phylogenetic analysis and the classification of H7N9 viruses As for HA and NA genes, the reference sequences used in our previous study [3] were used for the inference of phylogeny. As for the internal genes, all H9N2 virus genomes from 2006 were obtained from the Influenza Virus Resource [21] . Together with the 89 novel H7N9 viruses, phylogenetic trees of each internal gene were inferred using the maximum likelihood method under the GTRGAMMA model with 1,000 bootstrap replicates ( Supplementary Fig. 3 ), implemented in RAxML [22] . According to the bootstrap value (>75) and the branch length (>0.001), we classified the viral gene each into clades. All the accession codes of public sequences can be found in the Supplementary Table 6 . Genotypic assignment for the H7N9 viruses According to the classification of each internal gene, we applied the following rules to assign genotype. Genotype G0 was assigned for viruses if all internal genes fell into the main clade (clade 1.1). If strains have one internal gene different from G0 in the phylogenetic classification, we assigned them as genotype G1 and so on, with strains with all six internal genes different from G0 being assigned as G6. Within each of G1–G6 series, genotypes were further assigned (for example, G2.1) if any internal gene came from a different origin. The decimal number was sequentially assigned to each distinct genotype. Estimation of the global parameters The 92 NA gene sequences with collection dates were classified into four groups, Shanghai ( n =27), Jiangsu ( n =28), Zhejiang ( n =23) and other provinces ( n =14). The estimation of average within-province nucleotide diversity ( π w ) and between-province nucleotide diversity ( π b ) was as described in Bedford et al. [20] Briefly, , where n =4 provinces and π ( i,i ) refers to diversity (nucleotide substitutions per site) of sequence pair in the same province. And , where π ( i,j ) refers to diversity of sequence pair in different provinces. We estimated evolutionary dynamics and the NA genealogy using the Bayesian phylogenetic method implemented in BEAST v1.7.2 (ref. 26 ). The uncorrelated lognormal relaxed molecular clock was used to accommodate rate variation among lineages [27] . The HKY85 model [28] of nucleotide substitution was used to parameterize the mutational process, with equilibrium nucleotide frequencies taken from observed frequencies, and with homogeneous rates across sites. Posterior distributions of parameters were estimated by Markov chain Monte Carlo (MCMC) sampling. Samples were drawn every 10,000 steps over a total of 2.0 × 10 7 steps, with 2.0 × 10 6 steps removed as burn-in. The transition/transversion ratio κ was estimated to be 8.294 (95% confidence interval: 4.633–12.057). The rate of nucleotide substitution μ was estimated to be 2.373 × 10 −2 substitutions per site per year (95% confidence interval: 1.823 × 10 −2 –4.583 × 10 −2 substitutions per site per year). Coalescent estimation of migration rates To estimate coalescent parameters for each geographic region, we used an MCMC technique implemented in Migrate v3.3.0 (refs 22 , 29 ). The prior distribution of Θ and 2 Nm values was assumed to be exponential with a mean of 1, and mutational parameters were fixed in the analyses. To minimize the influence of sampling patterns on our results, we performed independent analyses of 100 resampled replicates. For each replicate, we randomly sampled 30 sequences with replacement from each region. For each of the 100 bootstrap replicates, 50 MCMC simulations were run for 6 × 10 6 steps each. The first 5 × 10 6 steps of each chain were removed as burn-in. Parameter values were sampled every 10 4 steps. Convergence was assessed visually and through comparison of chains using the Gelman-Rubin convergence statistic [30] . We combined the remaining samples from each chain to give a total of 5,000 samples for each of the resampled replicates. Genealogical inference We fixed Θ and 2 Nm at the values estimated in the previous analysis. We ran four MCMC chains for 2 × 10 8 steps each, of which the first 10 8 steps were removed as burn-in, with genealogies sampled every 10 5 steps. Accession codes Sequences deposited in GenBank: KF034884 to KF034891 , KF007041 to KF007080 , KF007001 to KF007016 , KF007105 to KF007120 , KF007137 to KF007152 , KF150613 to KF150620 . Sequences deposited in EpiFlu database: EPI460748 to EPI460755, EPI443632 to EPI443655, EPI460764 to EPI460779, EPI453647 to EPI453652. How to cite this article: Cui, L. et al. Dynamic reassortments and genetic heterogeneity of the human-infecting influenza A (H7N9) virus. Nat. Commun. 5:3142 doi: 10.1038/ncomms4142 (2014).